A phenylalanine rotameric switch for signal-state control in bacterial chemoreceptors Bacterial chemoreceptors are widely used as a model system for elucidating the molecular mechanisms of transmembrane signalling and have provided a detailed understanding of how ligand binding by the receptor modulates the activity of its associated kinase CheA. However, the mechanisms by which conformational signals move between signalling elements within a receptor dimer and how they control kinase activity remain unknown. Here, using long molecular dynamics simulations, we show that the kinase-activating cytoplasmic tip of the chemoreceptor fluctuates between two stable conformations in a signal-dependent manner. A highly conserved residue, Phe396, appears to serve as the conformational switch, because flipping of the stacked aromatic rings of an interacting F396-F396′ pair in the receptor homodimer takes place concomitantly with the signal-related conformational changes. We suggest that interacting aromatic residues, which are common stabilizers of protein tertiary structure, might serve as rotameric molecular switches in other biological processes as well. Chemotactic bacteria monitor and respond to their environment using specialized molecular machinery built around a two-component signalling system with enhanced capabilities [1] , [2] . Although chemotaxis systems in prokaryotes are diverse, their core components, extensively studied in the model organism Escherichia coli , are well conserved [3] . Chemotaxis systems have remarkable signalling properties, such as stimulus integration and amplification, stimulus sensitivity over a wide dynamic range, and sensory adaptation [4] . Chemoreceptors, known as methyl-accepting chemotaxis proteins, are central to these features [1] , [4] , [5] . E. coli chemoreceptors are transmembrane homodimers that carry sites of covalent modification that enable molecular memory [1] , [5] ( Fig. 1a ). Receptor dimers form trimers of dimers, which can contain receptors of different detection specificities ( Fig. 1b ). Receptor trimers recruit the cytoplasmic proteins CheA and CheW to form signalling teams, the minimal functional unit [6] , [7] , [8] . Receptor teams, in turn, assemble into higher order, hexagonal arrays [9] that impart highly cooperative responses to chemoeffector changes [10] . In isotropic chemical environments, receptor arrays activate the CheA kinase leading to phosphorylation of the response regulator CheY. Phospho-CheY binds to flagellar motors to promote clockwise flagellar rotation, which causes random changes in swimming direction. Increasing attractant levels deactivate CheA, promoting counter clockwise flagellar rotation, which produces forward swimming. Following an attractant-induced swimming change, the cell’s sensory adaptation system covalently modifies the signalling receptors to terminate the behavioural response: Methylation of specific glutamate residues in the receptor cytoplasmic domain (see Fig. 1 ), mediated by the methyltransferase CheR, enhances CheA activity; receptor demethylation, catalysed by the methylesterase CheB, reduces CheA activity. 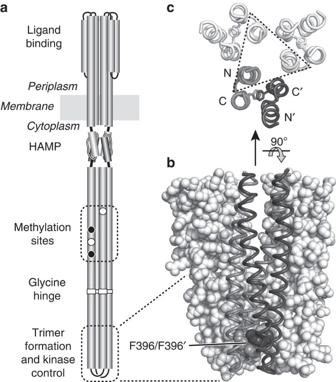Figure 1: Structure-function features of theE. coliserine chemoreceptor Tsr. (a) Cartoon of the Tsr homodimer. Cylindrical segments represent α-helical regions, drawn approximately to scale. The entire cytoplasmic portion below the HAMP domain comprises a four-helix, antiparallel, coiled-coil bundle. Methylation sites shown as black circles indicate glutamine (Q) residues; white circles represent glutamate (E) residues. The hairpin tip of the cytoplasmic bundle contains residues that promote interactions with other receptor molecules to form trimers of dimers and with the cytoplasmic CheW and CheA proteins to form ternary signaling complexes. (b) Tsr residues 350–430 in trimer-of-dimers association two dimers are shown space-filled (white), the third is shown in backbone trace with one subunit shaded grey and the other dark grey. The stacked F396 residues in the third dimer are shown space-filled. (c) Tsr residues 380–400 in trimer-of-dimers association, viewed from the membrane towards the tip. Backbone traces of the four helices in each dimer are shown, with the F396 residues indicated as sticks. Most of the trimer-stabilizing side-chain interactions (not shown) take place between tip residues in one N-terminal helix from each dimer (enclosed in the dashed triangle). Figure 1: Structure-function features of the E. coli serine chemoreceptor Tsr. ( a ) Cartoon of the Tsr homodimer. Cylindrical segments represent α-helical regions, drawn approximately to scale. The entire cytoplasmic portion below the HAMP domain comprises a four-helix, antiparallel, coiled-coil bundle. Methylation sites shown as black circles indicate glutamine (Q) residues; white circles represent glutamate (E) residues. The hairpin tip of the cytoplasmic bundle contains residues that promote interactions with other receptor molecules to form trimers of dimers and with the cytoplasmic CheW and CheA proteins to form ternary signaling complexes. ( b ) Tsr residues 350–430 in trimer-of-dimers association two dimers are shown space-filled (white), the third is shown in backbone trace with one subunit shaded grey and the other dark grey. The stacked F396 residues in the third dimer are shown space-filled. ( c ) Tsr residues 380–400 in trimer-of-dimers association, viewed from the membrane towards the tip. Backbone traces of the four helices in each dimer are shown, with the F396 residues indicated as sticks. Most of the trimer-stabilizing side-chain interactions (not shown) take place between tip residues in one N-terminal helix from each dimer (enclosed in the dashed triangle). Full size image Receptor ternary complexes operate as allosteric enzymes in equilibrium between two signalling states, kinase-on and kinase-off [1] , [11] . In E. coli , receptor outputs reflect the interplay of ligand-binding inputs with the methylation status of the sensory adaptation system [12] , [13] . In Tsr, the serine-detecting receptor of E. coli , the methylation sites and the kinase interaction region reside in the cytoplasmic carboxy-terminal signalling domain, comprising a 20 nm long, antiparallel, four-helix, coiled-coil bundle [14] ( Fig. 1a ). Mutagenesis studies have shown that glutamine replacements at the methyl-accepting glutamate residues mimic the signalling effects of methylation [15] . Thus, Q residues can simulate the fully methylated (kinase-on) receptor state (QQQQ), whereas E residues represent the fully demethylated (kinase-off) state (EEEE). Newly-synthesized wild-type receptor molecules contain glutamine residues at two of the four methylation sites in each subunit (QEQE) and have intermediate kinase activities until deamidated by the CheB methylesterase in preparation for subsequent CheR-mediated methylation [16] , [17] . A large body of theoretical, structural, biochemical and mutational evidence indicates that transmembrane signalling in E. coli receptors occurs through piston displacements of one transmembrane helix in the receptor dimer [18] , [19] , [20] , providing conformational control between the extracellular ligand-binding site and the cytoplasmic HAMP domain [21] , [22] ( Fig. 1a ). The HAMP domain, in turn, converts asymmetric piston input into a symmetric conformational output that modulates the packing stability of the methylation helices [23] . The subsequent kinase control mechanisms employed by the hairpin tip of the receptor ( Fig. 1a ), are not well understood. Structural and bioinformatics data suggest bending of the receptor four-helix bundle at the glycine hinge between the methylation sites and the signalling tip [24] , [25] , [26] ( Fig. 1a ). Stimulus-induced bending is consistent with anisotropy measurements of fluorescently labelled receptors in vivo [27] , [28] . Recent theoretical work also proposes bending as a signalling mechanism, although that bending involved a different region of the signalling domain [29] . On the other hand, crosslinking studies do not support either overall bending of the receptor or a relative piston motion between dimers within a trimer as a signalling mechanism [30] . Extensive genetic and biochemical experiments proposed that signals are conveyed between the adaptation region and receptor tip through oppositional changes in helix–helix packing [31] . Thus, key questions regarding signal transmission through the receptor molecule remain unanswered. In particular, what are the mechanisms by which conformational changes traverse a receptor dimer and influence kinase activity in the ternary signalling complex [1] ? An emerging signalling paradigm is that protein dynamics play an important role in signal transduction. Proteins fluctuate among many structural states on evolutionarily selected energy landscapes; stimulus inputs can transmit information by remodelling the dynamic landscape [32] . New methodologies provide insight into the dynamic properties of proteins at the atomic scale. Microsecond-range all-atom MD simulations have already yielded an unprecedented level of detail in such processes as protein folding [33] , [34] , mechanisms of voltage gating in ion channels [35] and signalling by EGFR kinase [36] and G-protein coupled receptors [37] . Here we describe a signal-dependent two-state conformational switch in the E. coli serine chemoreceptor Tsr revealed by long-duration (7 μs) all-atom MD simulations. We show that this switch is localized to the kinase-binding region of the receptor tip and manifests as alterations between gauche and trans conformations of Phe396, the single, most conserved residue in the chemoreceptor superfamily. Chemoreceptor structural asymmetry Although Tsr functions in trimer-of-dimer signalling teams, the very large trimers are impractical subjects for long-duration, all-atom MD simulations. Accordingly, we examined the dimeric Tsr signalling domain for signalling-related conformational states. In the crystal structure of the trimeric Tsr signalling domain, the two subunits of each dimer have non-equivalent structures [14] ( Fig. 1c ). The amino-terminal cytoplasmic helix of one subunit (hereafter designated the N helix) makes the majority of trimer-stabilizing contacts, whereas its counterpart in the other subunit (the N′ helix) lies on the periphery of the trimer ( Fig. 1c ). The CheW coupling protein and the CheA kinase probably interact with exposed binding determinants in the N′ helices of the trimers to form ternary signalling complexes [7] , [38] . The inherent structural asymmetry of the signalling domain subunits in a Tsr dimer, which is likely enforced from the trimeric crystal structure, in the absence of other protein-protein contacts, should eventually dissipate over an extended MD simulation. However, despite the structure being equilibrated with the rest of the simulation system, the N/C and N′/C′ subunits remained distinctly different, presumably reflecting their different roles in the ternary signalling complex. The kinase-binding tip of the receptor is highly dynamic We performed 2 μs, all-atom MD simulations of the full-length Tsr signalling domain (residues 263–519) in three modification states, each corresponding to a distinct signalling activity [15] ( Supplementary Fig. S1 ). The QQQQ receptor mimics the fully methylated form and activates the CheA kinase (ON state); the EEEE receptor is fully unmethylated and fails to activate the kinase (OFF state) [12] , [13] . A simple two-state allosteric model of kinase regulation [39] predicts that the half-modified QEQE form of the receptor should be in equilibrium between these alternative signalling states. The internal backbone dynamics of a protein can be inferred from MD trajectories using the ‘model-free’ formalism proposed by Lipari-Szabo [40] . The generalized order parameter S 2 , calculated from the backbone NH bond vector, carries information about the flexibility of the structure. High values of the order parameter (that is, close to 1) indicate less flexibility. Our simulation runs revealed strikingly similar Tsr backbone dynamics in all three modification states ( Supplementary Fig. S2 ). Overall, Tsr had a relatively rigid backbone ( S 2 >0.9) with two segments of higher flexibility. A region containing two conserved glycines (Gly340 and Gly341), part of a so-called glycine hinge [41] , had a lower order parameter than adjacent regions ( Supplementary Fig. S2 ), in agreement with previous experimental and computational data [24] , [25] , [31] . However, analysis of bending properties along the receptor structure did not show any increased bending propensity at the glycine hinge ( Supplementary Fig. S3 ). The most dynamic part of the receptor, in all three modification states, was its hairpin tip (residues 383–397), which contains the principal determinants for CheA binding [42] , [43] . Two signal-dependent conformations at the receptor tip To further investigate the highly dynamic receptor tip, we applied a measure of the root mean squared deviation (r.m.s.d.) of each coordinate frame against the first frame in all simulations. Analysis of the r.m.s.d. over time showed that in all three signalling states, the tip oscillated between two conformations ( Supplementary Fig. S4 ). Visual inspection of the trajectories suggested that the difference between the two conformations was likely due to the relative displacements of helices in the chemoreceptor four-helix bundle. To quantify these effects, we measured distances between alpha carbons in the four-receptor helices at consecutive single-residue levels. In all simulations, the distances between helices C–C′, N–N′, C–N and C′–N′ remained constant, whereas distances between helices C–N′ and N–C′ oscillated between two conformations that differed by ~3 Å ( Fig. 2 and Supplementary Fig. S5 ). Furthermore, as the distance between C–N′ became smaller, the distance between C′–N in the same bundle-packing layer became larger, and vice versa ( Supplementary Fig. S6 ). This synchronous behaviour suggests a concerted movement of this region of the receptor molecule. Finally, our numerical analyses showed that there is a preferential conformation for each signalling state. During the 2 μs simulations, the QQQQ and EEEE receptors mostly assumed opposite conformations ( Fig. 2 ). Remarkably, the QEQE receptor oscillated between the two conformations, consistent with a two-state model of chemoreceptor signalling [1] , [39] . 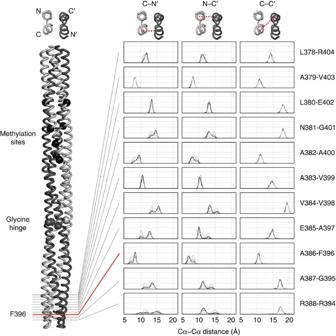Figure 2: Two stable conformations at the chemoreceptor tip. Left: Backbone structure of residues 263–519 in the hairpin tip of the Tsr dimer. The N helix of the light grey subunit is located at the trimer axis (seeFig. 1). Alpha carbon atoms mark the locations of the methylation sites (residues 397, 304, 311, 493) and the glycine hinge (residues 340, 341, 439). The side chains of residues F396 and F396′ are shown as sticks. Right: Distance distributions over the course of the MD simulations between helices C–N′, C′–N and C–C′ of the Tsr structure at a single residue-pair level for each methylation state: QQQQ (dark grey), QEQE (black) and EEEE (light grey). Figure 2: Two stable conformations at the chemoreceptor tip. Left: Backbone structure of residues 263–519 in the hairpin tip of the Tsr dimer. The N helix of the light grey subunit is located at the trimer axis (see Fig. 1 ). Alpha carbon atoms mark the locations of the methylation sites (residues 397, 304, 311, 493) and the glycine hinge (residues 340, 341, 439). The side chains of residues F396 and F396′ are shown as sticks. Right: Distance distributions over the course of the MD simulations between helices C–N′, C′–N and C–C′ of the Tsr structure at a single residue-pair level for each methylation state: QQQQ (dark grey), QEQE (black) and EEEE (light grey). Full size image Residue Phe396 governs conformational changes at the tip One of the advantages of the all-atom MD approach is the possibility of tracing the individual behaviour of amino-acid residues in proteins. Accordingly, we measured side-chain χ 1 dihedral angles (between the N–Cα–Cβ−Cγ atoms) for all residues in the four-helix receptor bundle. The only significant variation correlated with the helix displacement was the behaviour of residue Phe396 at the receptor tip, which forms a Phe-Phe stacking interaction between the C′–C helices of the dimer ( Supplementary Fig. S7 ). The χ 1 dihedral angle of the Phe396 side chain changed periodically during simulation runs from gauche ( χ 1 ~−60°) to trans ( χ 1 ~180°), which causes the aromatic rings of interacting Phe396 and Phe396′ simultaneously flipped by 180° significantly changing their local environment ( Fig. 3a and Supplementary Movies 1 and 2 ). The Phe396 switching events coincided with the conformational changes observed in the C–N′ and N–C′ helix pairs ( Fig. 3b ). The Pearson’s product–moment correlation between the time evolution of the χ 1 dihedral angle and the distance between C–N′ in each state were as follows: r =−0.75 for QQQQ, r =−0.82 for QEQE and r =−0.79 for EEEE (two-tailed t -test P -value<2.2 × 10 −16 for all coefficients). The preference for gauche / trans or trans/gauche arrangements in each receptor modification state was evident over the course of the simulation runs ( Fig. 3c ): The distribution of χ 1 values for the QQQQ receptor was exactly opposite that for the EEEE receptor; the distribution for the QEQE receptor state had more balanced proportions of gauche and trans conformations. 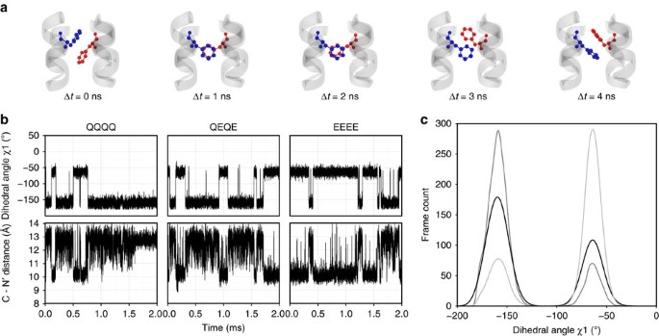Figure 3:Gauche-transswitch of the Phe396 side-chain. (a) Time lapse of thegauche-transswitch. (b) Time evolution of the dihedral angleχ1of Phe396 in the helix C (blue in panela) and the distances between the helices C–N′ for each simulation and methylation state. (c) Distribution of the dihedral angleχ1during simulations in three methylation states: QQQQ (dark grey), QEQE (black) and EEEE (light grey). Figure 3: Gauche-trans switch of the Phe396 side-chain. ( a ) Time lapse of the gauche-trans switch. ( b ) Time evolution of the dihedral angle χ 1 of Phe396 in the helix C (blue in panel a ) and the distances between the helices C–N′ for each simulation and methylation state. ( c ) Distribution of the dihedral angle χ 1 during simulations in three methylation states: QQQQ (dark grey), QEQE (black) and EEEE (light grey). Full size image Phe396 is the most conserved residue in chemoreceptors One of the central paradigms of evolutionary biology is that residues conserved over long evolutionary distances are important for the function of the protein, either by contributing to enzymatic activity, to a docking site for an interacting protein or to a stable tertiary structure [44] . The chemoreceptor’s kinase-binding subdomain is highly conserved, owing to the multifaceted nature of its interactions [25] . To determine the conservation level of Phe396 within this subdomain, we collected and aligned 7,809 non-redundant sequences of the chemoreceptor signalling domain from all complete bacterial and archaeal genomes in the MiST database [45] as of August 2012. This multiple sequence alignment revealed that Phe396 is the most conserved residue in the entire chemoreceptor protein family ( Supplementary Table S1 ). The universal presence of this amino acid in the signalling tip of chemoreceptor molecules suggests that Phe396-Phe396′ gauche-trans switching is critically important for proper chemoreceptor function. To explore the functional importance of Phe396 in Tsr, we constructed a complete set of mutant receptors with amino-acid replacements at this residue and tested their ability to mediate a chemotactic response to serine on tryptone soft agar plates ( Fig. 4 ). All mutant receptor proteins had normal intracellular expression levels, consistent with a near-native structure. However, none of the mutant receptors mediated a wild-type chemotactic response. Ten were fully defective; the other nine F396 amino-acid replacement mutants mediated aberrant chemotactic responses with at most half of the wild-type functionality ( Fig. 4 ). These results confirm that Phe396 is, indeed, important for proper Tsr function. No other amino acid can serve the same purpose at this position in the receptor molecule’s signalling hairpin tip. 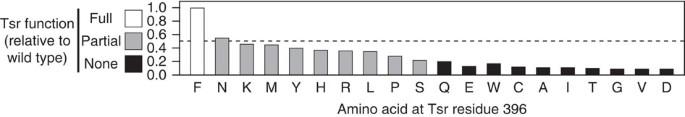Figure 4: Chemotactic function of Tsr-F396 amino-acid replacement mutants. Chemotactic ability of cells carrying a mutant Tsr as their only chemoreceptor was evaluated by the size and morphology of their colonies on tryptone semi-solid agar plates after incubation for 8 h at 30 °C. Colony sizes were normalized to that of a wild-type Tsr control colony on the same plate. Mutant receptors with partial function (grey bars) produced colonies with a ring of chemotactic cells at their periphery, but with smaller diameters than the wild-type control. Figure 4: Chemotactic function of Tsr-F396 amino-acid replacement mutants. Chemotactic ability of cells carrying a mutant Tsr as their only chemoreceptor was evaluated by the size and morphology of their colonies on tryptone semi-solid agar plates after incubation for 8 h at 30 °C. Colony sizes were normalized to that of a wild-type Tsr control colony on the same plate. Mutant receptors with partial function (grey bars) produced colonies with a ring of chemotactic cells at their periphery, but with smaller diameters than the wild-type control. Full size image The ‘new view’ of protein allostery proposes that proteins populate ensembles of conformations. Inputs, such as ligands or covalent modifications, remodel the conformational landscape to bias the population distribution towards a particular signal output [32] . In this MD study, we found that the kinase-activating tip of the E. coli Tsr chemoreceptor is highly dynamic and fluctuates between two stable conformations. We suggest that the conformation favored by the CheA-activating QQQQ form of the receptor corresponds to the kinase-on signal state; the alternative conformation, preferentially populated by the CheA-deactivating EEEE form of the receptor, represents the kinase-off signal state. The QEQE form of the receptor populates both conformational states, consistent with its intermediate level of CheA activation observed experimentally. An invariant tip residue, Phe396, appears to serve as a molecular switch for accessing these two receptor signalling conformations. F396 forms a stacking interaction with F396′ from the other subunit in the receptor homodimer. In the MD simulations, Phe-Phe flipping events occurred synchronously with the signalling-related conformational changes at the receptor tip. MD simulations were carried out on an isolated receptor dimer, where monomers appear to be symmetric, which poses a problem for interpreting our results: upon a 180° rotation about the dimer axis, the preferable conformational state of the QQQQ structure would be identical to that of the preferable state of the EEEE structure. However, there was an inherent asymmetry in the starting configuration of the dimer, likely enforced from the trimer contacts in the crystal structure from where the starting coordinates came. This asymmetry is maintained during simulation, although we anticipate that during a longer simulation time, it should dissipate. Key conformational changes, apart from the Phe-Phe flipping, involve the C–N′ and N–C′ contacts. Our model assumes that these contacts are also asymmetric in the isolated dimer coming from the trimer structure, because of their distinct roles in the trimer. What is the exact nature of anticipated subtle conformational differences between these contacts remains unknown. With a future increase in computing power, longer simulations of the entire trimer of dimers will be able to address this problem directly. To further verify the unique nature of the Phe396 residue revealed by our MD simulations and comparative genomics, we have carried out a survey of all possible amino-acid replacements at F396. We found that no other amino acid at this residue position could replicate wild-type Tsr function. Amino acids with an acidic (D, E), small hydrophobic (G, A, V, I), polar (T, Q) or very large (W) side chain disrupted function entirely. These replacements may prevent Tsr from accessing one or both of the postulated signalling conformations. Amino acids with a basic (H, K, R), small polar (P, S, N) or large hydrophobic (L, M) side chain impaired, but did not fully abrogate, function. Conceivably, these replacements might preferentially stabilize one of the signalling conformations, biasing receptor output towards the kinase-on or kinase-off state and thereby attenuating stimulus responses. Even tyrosine, whose side chain most closely resembles that of phenylalanine, severely affected Tsr function, emphasizing the unique signalling role played by F396. Cysteine-directed crosslinking studies of the aspartate chemoreceptor Tar, a Tsr paralog, (F396 in Tsr corresponds to F394 in Tar), showed that a disulphide bond between F394C and F394C′ in the Tar dimer locked receptor output in the kinase-activating mode, whereas reduction of the disulphide bond allowed Tar–F394C to downregulate kinase activity in response to aspartate [31] , [46] , [47] . The Tar–F394C receptor was the only one among many cysteine replacement constructs in which a disulphide bond allowed high kinase activity [31] , [46] , [47] . According to our model of F396 action, a disulphide bond between subunits at this position must trap the receptor dimer in the kinase-on conformation. Connecting the current atomic level descriptions of dynamic behaviours in a receptor dimer to their signalling roles in trimer-of-dimer teams and higher-order arrays remains the grand challenge. While microsecond scale simulations are capable of capturing many physiologically relevant dynamic changes in the protein, large-scale conformational rearrangements may occur more slowly. However, the structural asymmetry imposed upon receptor dimers by their trimer-of-dimer organization most likely potentiated the signalling-related conformations observed in our MD simulations. Accordingly, extrapolation of those structural shifts to the trimer-of-dimers geometry, which is universally conserved in bacteria [9] , provides new insights into the chemoreceptor signalling mechanism ( Fig. 5 and Supplementary Movie 3 ). We propose that the N helices of each receptor, which provide most of the trimer-stabilizing interactions between tips of the dimers, function as conformational fulcrums for signalling-related changes in the trimer. The N helices maintain inter-receptor contacts throughout the signalling cycle, whereas the C, N′ and C′ helices shift in unison toward (kinase-on) or away from (kinase-off) the trimer axis ( Fig. 5 ). These motions probably modulate kinase activity by manipulating CheA domains associated with the receptor helices at the periphery of the trimer [48] . 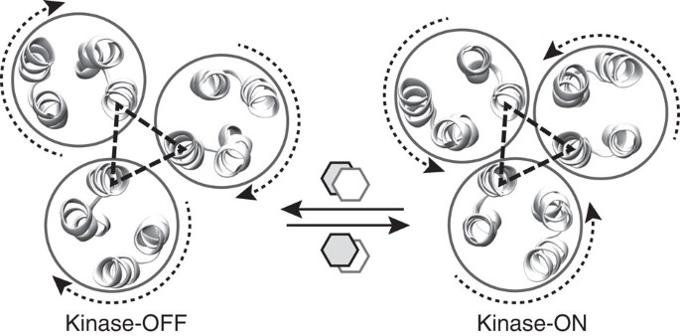Figure 5: Model for modulation of kinase activity by receptor trimers of dimers. Shown are cross-section views of the four-helix bundles near the signaling tip of receptor dimers. The N helices of three receptors, connected by dashed triangles, interact to form trimers of dimers that remain associated throughout the receptors’ signaling cycle. The model proposes two signalling conformations at the receptor tip that are stabilized by alternative stacking arrangements of Phe396 residues in each receptor dimer. The signalling states differ by concerted motions of the outer helices in each dimer, which make binding contacts to the CheW coupling protein and the CheA kinase (not shown). To access the kinase-off state, the N and C′ helices move further apart and the C and N′ helices move closer together. To access the kinase-on state, those motions are reversed. The proposed dynamics of the trimer of dimers is shown inSupplementary Movie 3. Figure 5: Model for modulation of kinase activity by receptor trimers of dimers. Shown are cross-section views of the four-helix bundles near the signaling tip of receptor dimers. The N helices of three receptors, connected by dashed triangles, interact to form trimers of dimers that remain associated throughout the receptors’ signaling cycle. The model proposes two signalling conformations at the receptor tip that are stabilized by alternative stacking arrangements of Phe396 residues in each receptor dimer. The signalling states differ by concerted motions of the outer helices in each dimer, which make binding contacts to the CheW coupling protein and the CheA kinase (not shown). To access the kinase-off state, the N and C′ helices move further apart and the C and N′ helices move closer together. To access the kinase-on state, those motions are reversed. The proposed dynamics of the trimer of dimers is shown in Supplementary Movie 3 . Full size image Small signalling-related conformational changes within the trimer contact region may lead to larger motions in other regions of the receptor dimers. The glycine hinge, for example, identified by previous experimental [24] , [26] and computational [25] studies, was suggested as a specific site for receptor bending, which could account for proposed splaying motions of the dimers [27] , [28] . Our MD results indicated that this region of the receptor was flexible, but provided no evidence for preferential bending at the glycine hinge. Although our simulations cannot identify the specific mechanism for transmitting structural influences between the methylation sites and receptor tip, in the energy landscape view of protein signalling [32] , it seems unlikely that the transmission mechanism involves a simple overall motion, such as bending at the glycine hinge. Instead, ligand binding and methylation probably change the receptor’s local energy landscape, thereby altering its range of sampled conformations. Excursions into newly allowed regions of the local conformational space would in turn influence the energy landscape of neighbouring regions. These conformational changes could be translated into a variety of mechanistic motions of different amplitudes in different parts of the structure: bending, torsion, vertical displacements and variations in helix packing. Some important structural shifts, likely to occur on the low-microsecond time scale, might be too complex to be identified by current MD methods, but should yield to new, more powerful experimental and computational approaches. The key signalling role of Phe396 in bacterial chemoreceptors implies that buried and paired aromatic residues, which are common stabilizers of protein tertiary structure [49] , might serve as conformational switches in other signalling systems. For example, recent MD experiments suggested that Phe-Phe and Phe-Trp stacking interactions might serve as conformational switches in HAMP domains [50] and seven transmembrane receptors [51] . We expect that as long MD simulations become more accessible, such rotameric aromatic switches will be discovered in many similar systems. Mutant isolation and functional characterization To assemble a full set of amino-acid replacements at Tsr residue 396, we performed all-codon QuikChange mutagenesis [8] using as template pPA114 (ref. 52 ), a plasmid that confers chloramphenicol resistance and carries wild-type tsr under inducible salicylate control. We verified all mutations by sequencing the entire tsr coding region. To test the function of mutant receptors, we introduced mutation-bearing plasmids into the receptorless strain UU2612 [Δ aer -1 Δ( tar - tap ) 4530 Δ tsr - 5547 Δ trg - 4543 ] [11] and assayed individual transformants for serine chemotaxis at 30 °C in tryptone soft agar plates [53] containing 12.5 μg ml −1 chloramphenicol and 0.6 μM sodium salicylate. In these assays, pKG116 (ref. 52 ), a relative of pPA114 with no tsr gene, served as a negative control. Expression levels of mutant Tsr proteins were determined in E. coli K12 strain UU2610, which lacks che CheR and CheB enzymes, to prevent adaptational modifications to the receptor molecules. Cells were grown in tryptone broth (10 g l −1 tryptone, 5 g l −1 NaCl) to mid-exponential phase, then concentrated and lysed by boiling in SDS sample buffer. Cell extracts were analysed by electrophoresis in SDS-containing 7% polyacrylamide gels and Tsr bands were visualized by immunoblotting with a polyclonal rabbit antiserum (1:1,500 dilution) directed against Tsr residues 290–470 (ref. 11 ). Bioinformatics We retrieved 12,498 chemoreceptor sequences from complete genomes in the MIST database as of August 2012 (ref. 45 ). Using previously described hidden Markov models [25] , the chemoreceptors were classified and separated into different files according to their heptad classes using HMMER software [54] . Sequences that did not match any heptad class were excluded from analysis. The methyl-accepting chemotaxis protein signal model from the Pfam database [55] was used to extract protein regions corresponding to the signalling domain. Sequences in each file were aligned using MAFFT [56] , excluding those that were more than 97% identical or incomplete. Multiple sequence alignments of each heptad class were trimmed to include only eight heptads (N04 to C04) adjacent to the hairpin turn (a total of 57 residues, D363 to S419 in Tsr protein). The sequence logo showing the information content measured as entropy (information content in bits) and the amino-acid distribution in each position in the alignment were generated using the Weblogo software [57] . MD simulation system We began with atomic coordinates for residues 263–519 of the Tsr dimer that were based on the X-ray crystal structure of the Tsr signalling domain in the QQQQ modification state (PDB code: 1QU7) [14] . The model approximately corresponds to the signalling domain boundaries [14] , [25] . The structure was embedded in water, tip3p, neutralized and supplemented with 5 mM NaCl. The total simulation system contained 144,647 atoms in a 90 × 90 × 182 Å 3 periodic box. To keep the structure in place during the simulations a 50 kcal mol −1 Å −2 restrain was placed in the backbone of the residues 263 and 519 and a 25 kcal mol −1 Å −2 restrain was placed in the backbone of the residues 264 and 518. MD simulations A 50 ns simulation with the MD engine Desmond 2.4 (ref. 58 ) was performed on a Linux cluster using 512 nodes for pre-equilibration of the system in NPT ensemble with Berendsen thermostat at 300 K constant temperature and 1 atm pressure. The system was then transferred to the 512 node, special-purpose supercomputer Anton [59] , where a 1-μs simulation was performed to assure equilibration of the entire structure. The structure of the last frame of this simulation was mutated in silico to change the methylation states of the structure: Q304E and Q493E to build the QEQE structure and Q297E, Q304E, Q311E and 493E to build the EEEE structure. Water molecules and ions were added as needed to restore minor changes in density and to neutralize the system. Local minimization was performed for eight steps in the mutated side chains on Maestro 9.1 (Schrodinger). The velocities were initialized using Desmond 2.4 prior to the transfer to Anton. Each of the three production simulation was 2 μs long. All simulations were performed using the CHARMM27 forcefield, NPT ensemble, 300 K, 1 atm and Berendsen integrator. Long-range electrostatics interactions used Gaussian split Ewald with a 64 × 64 × 64 FFT mesh [60] . The 64 grid points over 220 Å length could lead to errors during the computation of forces. However, this is a hardware limitation of Anton, and we increased the cutoff of electrostatics interactions to compensate for this hardware limitation. During the preparation of the system, a short simulation was performed to test the accuracy of force computation on Anton. The programme measures the root mean squared (r.m.s.) force error, defined as the r.m.s. error in the force on all particles divided by the r.m.s. force. The simulation is only cleared for execution if the relative r.m.s. force error is below 0.001, which is considered sufficiently accurate for biomolecular MD simulations on Anton [59] . Consequently, we used the smallest possible cutoff for short range interactions and van der Waals at 16.75 Å that guarantees best performance with r.m.s. force error below 0.001, with sufficient accuracy. The simulations time step was 1 fs and respa scheme 1:1:3 that is, long-range electrostatic interactions were calculated every third step. Calculation of the order parameter The current methodology to calculate order parameter assumes that the frames of the simulations have been aligned to a reference frame to avoid coupling between rotational and/or translational movements and the internal motions. This procedure works well for globular proteins but fails in the case of multidomain structures and/or largely anisotropic structures such as the chemoreceptor. To overcome this problem, we developed a procedure to minimize the problem of frame alignment in anisotropic structures: local alignment per residue protocol. As the internal correlation function is calculated for each residue, each frame of the simulation is aligned to the reference frame using only a selection of atoms within a certain distance from the target residue. This custom selection of atoms per residue is insensitive to translational/rotational motions between parts of the structure. Here we used 30 Å cutoff. The result is robust to cutoff variations. The order parameter is defined as [40] , [61] : where C I (∞) is the internal correlation function when t →∞ Also, t and τ scans over the sequence of frames, is the unit vector pointing along the backbone 15 N–H bond. P 2 ( x )= is the second Legendre polynomial. The equation (1) requires a convergence of C I ( t ) as t increases. To verify the convergence, we calculate the correlation function as: then we define C tail as the average of the values of the last 0.5 ns of the correlation function. Convergence is assumed if <0.005 as previously proposed [62] . If there is no convergence, the order parameter is considered null. Trajectory analysis Dihedral angles and alpha carbon distances were extracted from the trajectories by custom python scripts using the MD toolkit MD Analysis v0.7.5 (ref. 63 ). Correlation function between the time series of dihedral angle and helix–helix distances (alpha carbon distances) were calculated using the ‘cor’ function from R statistical package v2.14.1. Histograms and time series were plotted with ggplot2 package [64] for R. Figures and movies were made using VMD 1.9.1 (ref. 65 ) that was also used for visual analysis of the trajectories and r.m.s.d. measurements. Calculation of the average bending angle To measure local bending properties in the chemoreceptor we pair equidistant residues of the center of the harping turn of the chemoreceptor (residue E391) and call it a residue layer. For example, the tenth residue from the center of the harping turn E391 towards the N-terminus is N381, which is paired to the tenth residue towards the C-terminus—G401—to form the E391-G401 layer. The angle between the largest component of the principal axis of inertia calculated for the alpha carbons of the four layers above the target layer and below the target layer is then denoted as a bending angle ( Supplementary Fig. S8 ). The calculations were performed using the function ‘measure inertia’ from VMD 1.9.1 (ref. 65 ). This strategy aims to minimize coupling between other movements, such as shear, torsion or stretching that might appear as bending, by cumulative bending of adjacent layers in a given frame. A time series of the bending angle was extracted for each layer and averaged over time for each production simulation. How to cite this article: Ortega, D. R. et al. A phenylalanine rotameric switch for signal-state control in bacterial chemoreceptors. Nat. Commun. 4:2881 doi: 10.1038/ncomms3881 (2013).